Proximity of iron pnictide superconductors to a quantum tricritical point In several materials, unconventional superconductivity appears nearby a quantum phase transition where long-range magnetic order vanishes as a function of a control parameter like charge doping, pressure or magnetic field. The nature of the quantum phase transition is of key relevance, because continuous transitions are expected to favour superconductivity, due to strong fluctuations. Discontinuous transitions, on the other hand, are not expected to have a similar role. Here we determine the nature of the magnetic quantum phase transition, which occurs as a function of doping, in the iron-based superconductor LaFeAsO 1– x F x . We use constrained density functional calculations that provide ab initio coefficients for a Landau order parameter analysis. The outcome is intriguing, as this material turns out to be remarkably close to a quantum tricritical point, where the transition changes from continuous to discontinuous, and several susceptibilities diverge simultaneously. We discuss the consequences for superconductivity and the phase diagram. One of the most fascinating open problems in condensed matter physics is the appearance of unconventional superconductivity close to a quantum critical point (QCP), a zero-temperature phase transition driven by a control parameter like pressure, charge-doping or magnetic field. The interplay between a T =0 quantum phase transition and superconductivity is well documented in heavy fermions [1] , [2] , [3] and is suspected to have an important role in cuprates [4] , [5] , [6] , [7] , [8] and iron-based superconductors [9] , [10] , [11] , [12] . The conventional wisdom is that as the system is tuned close to the QCP the main effect of critical fluctuations is to act as the pairing glue, responsible for the superconducting phenomenon. [6] , [7] , [13] She and Zaanen [14] have recently suggested to shift the attention from the pairing glue to the pairing susceptibility. This is an insightful point of view because, at quantum criticality, the system has a large ground state degeneracy, and superconductivity is a natural candidate to remove this degeneracy [3] , [15] , [16] . Thus, the enhanced superconductivity close to a QCP can be seen as the effect of an enhanced pairing susceptibility as the QCP is approached, rather than the effect of an enhanced interaction. Layered superconductors based on Fe–As planes with a transition temperature up to 26 K in LaFeAsO 1− x F x and exceeding 50 K in related compounds have appeared as a new test ground for QCP ideas. 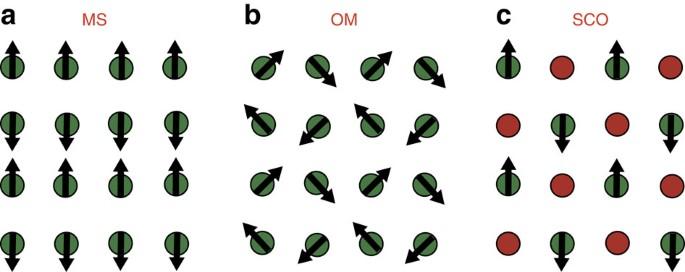Figure 1: Magnetic orders. Competing magnetically ordered states in LaOFeAs. (a) is the well-known magnetic stripe phase. (b) is the orthomagnetic phase with the nearest neighbours magnetic moments at right angles and (c) is the spin-charge ordered phase. Neutron scattering experiments [17] have shown that long-range magnetic stripe order as depicted schematically in Figure 1a develops in the FeAs planes of the parent compound, as predicted by density functional theory [18] . On doping the magnetic order is suppressed and disappears at zero temperature at a QCP. The phase diagram is strikingly similar to that of heavy fermions where the QCP is inside or on the edge of the superconducting dome, which strongly suggests that QCP physics has a major role. [9] , [10] , [11] , [12] Figure 1: Magnetic orders. Competing magnetically ordered states in LaOFeAs. ( a ) is the well-known magnetic stripe phase. ( b ) is the orthomagnetic phase with the nearest neighbours magnetic moments at right angles and ( c ) is the spin-charge ordered phase. Full size image Empirically, the magnetic 'thermal' transitions indeed show two types of behaviour [19] , [20] . In some compounds, typical of the so-called 122 family, like, for example, SrFe 2 As 2 , the transition is of first order, whereas in compounds of the 1111 family (like LaFeAsO), it appears as second order. This gives a first indication that the iron pnictides are close to a tricritical point, that is, a point in the temperature– x plane, where x is a non-thermal parameter, and where the nature of the transition changes from first to second order. It is conceivable, in principle, that, by changing two non-thermal parameters, the tricritical point can be driven to low or even zero temperature, giving rise to a quantum tricritical point (QTCP) where a wealth of unconventional quantum critical phenomena is expected to occur. [21] , [22] , [23] Although it seems unlikely that a material in which one non-thermal parameter is controlled can be tuned to a QTCP, as a matter of fact, in recent years, materials have emerged which appear to be surprisingly close to a QTCP, and accordingly show unexpected phenomena. For example, spiral ferromagnetism in ultraclean MnSi appears at a second-order phase transition at ambient pressure with a Curie temperature T c that decreases monotonically with pressure and turns into a first-order phase transition very close to the critical pressure p c , where T c is driven to zero. The proximity to a QTCP can be responsible for the anomalously broad and yet not-well-understood region of partial order and non-Fermi-liquid behaviour found for pressure above p c [24] , [25] . It is believed that, in this material, the lack of inversion symmetry suppresses superconductivity and other exotic orders have been proposed to emerge [26] , [27] , [28] . QTCP behaviour has also been proposed to occur in Sr 3 Ru 2 O 7 (ref. 29 ) and in some heavy-fermion anti- ferromagnets. In the latter case one can tune to the QTCP using both a uniform magnetic field and pressure. As stressed in ref. 21 , a remarkable property of QTCP's is that not only the order parameter fluctuations diverge but the susceptibility of the conjugate variables of the control fields (like the uniform magnetic susceptibility in the latter example) diverge as well. The nature of the magnetic phase transition in iron pnictides can be determined from a Landau order parameter analysis, if the coefficients that appear in the expansion are known. Here, by identifying all possible and relevant magnetic phases [30] close to a potential tricritical point, we determine all the coefficients of the Landau theory in LaFeAsO as a function of doping from first principles, computing total energies in a constrained density functional approach [31] within the local-density approximation (LDA) [32] , [33] , [34] . Using this approach, we find that LaFeAsO is surprisingly close to a QTCP that will strongly affect the superconducting and normal state properties. The resulting effective field theory [11] shows that, at this critical point, an Ising and a continuous order parameter vanish concomitantly. A structural transition must, therefore, be very close to the magnetic one, as indeed is found in the experimental phase diagram of LaFeAsO [35] . Landau Theory We can construct the Landau theory of magnetic order in iron-based superconductors on the basis of the assumption that the dominant magnetic instability of FeAs planes is at momentum ( π , 0) and (0, π ) where we use a notation with a single Fe per unit cell and take the Fe–Fe distance a ≡1. A previous study [30] has shown that a complete characterization of the physics around a potential QTCP in FeAs planes requires consideration not only of the well-known magnetic stripe phase (MS) with ordering wave vector ( π , 0) or (0, π ) ( Fig. 1a ) but also of a phase in which magnetic moments at nearest neighbour sites are at right angles, termed orthomagnetic (OM) ( Fig. 1b ), and a phase in which the real space magnetization is zero in one sublattice and forms an antiferromagnetic structure in the other sublattice ( Fig. 1c ). This phase has spin and charge order (SCO) and is reminiscent of the charged stripe phase in cuprates. Consistently with the expected generality of a Landau analysis, these states indeed appear as low-lying energy phases in microscopic computations [36] , ab initio [37] , [38] and density-matrix renormalization group studies [39] . The Landau free energy, specialized for the three possible ordered phases, as a function of their total magnetization M T reads We keep up to the sixth power of the magnetization to account for second- and first-order phase transitions. Knowledge of the seven coefficients appearing in equation (1) completely determines the Landau free energy functional around the tricritical point (except for gradient terms) [30] . Constrained density functional Density functional theory calculations within LDA are a good starting point to determine a bare Landau energy functional as they provide reasonably good estimates of ground state energy differences and of their derivatives as demonstrated, for example, by frozen phonon computations in strongly correlated systems [40] . Here we perform analogous 'frozen magnetization' computations to obtain the energy of the different phases and compute the Landau parameters (Methods). 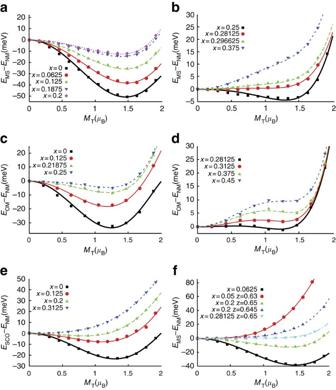Figure 2: Constrained LDA energies. Energy per Fe for the MS (a,b), the OM phase (c,d) and the SCO phase (e) as a function of the Fe magnetic moment for different doping concentrationx. The points are the results of LDA calculations whereas the continuous lines are fits using equation (1). (f) Energy per Fe for the MS phase for different values of thezcoordinate of the As in the unit cell. In Figure 2 we show the total energy per Fe ion for the three competing phases as a function of the local Fe magnetic moment M T and different doping concentrations. The zero of the energy is taken at the M T =0 state. The points are the LDA data and the lines the Landau fits. In general, we find that the latter provides an excellent fit to the data, even when M T is not small. For the MS in the undoped case ( x =0), the energy curve shows a clear deep minimum for M T ~1.5 μ B ( Fig. 2a ). By increasing the F-doping, the minimum moves to slightly lower magnetization values and eventually disappears for x >0.3 ( Fig. 2b ). The energy is extremely flat close to the critical point with the large moment state almost degenerates with the zero magnetic state and without the appearance of a noticeable energy barrier. This behaviour already indicates proximity to a QTCP and an anomalously 'soft' magnetism at the transition. For the OM state (c.f. Fig. 2c and d ), the behaviour has a more pronounced first-order character. The metastable minimum persists up to large dopings with a sizeable barrier separating the large magnetization state from the low-magnetization state. Finally, for the SCO state ( Fig. 2e ), the evolution is that of a typical second-order phase transition. We notice that the flatness of the energy landscape close to the critical point is a big obstacle for the numerical convergence of conventional unconstrained LDA computations, which is overcome by our constrained calculations. Figure 2: Constrained LDA energies. Energy per Fe for the MS ( a , b ), the OM phase ( c , d ) and the SCO phase ( e ) as a function of the Fe magnetic moment for different doping concentration x . The points are the results of LDA calculations whereas the continuous lines are fits using equation (1). ( f ) Energy per Fe for the MS phase for different values of the z coordinate of the As in the unit cell. Full size image Ab-initio Landau parameters From the statistical mechanics point of view, the LDA is a mean-field theory. Thus in the second-order region of the phase diagram, at the LDA level, one should, and indeed does, find classical critical exponents. The order parameter as a function of a non-thermal parameter vanishes as | x–x α | β with β LDA =1/2 far from the tricritical point and β LDA =1/4 at the tricritical point. The coefficient of the quadratic term corresponds, irrespective of the phase under consideration, to the inverse of the susceptibility of the non-magnetic phase at momentum ( π , 0) or (0, π ). Thus, a single parameter α appears in equation (1). As a consistency check, we allowed for different values of α in the fits and found that indeed α converges to practically the same values as a function of doping except for x ~0 and 0.5 where higher order terms in the expansion become important ( Fig. 3a ). The vanishing of α at a critical doping x α determines the limit of stability of the paramagnet coming from large x . For the experimental lattice constants, we find α ~0.26( x–x α ) eV/ μ B 2 with x α =0.27. 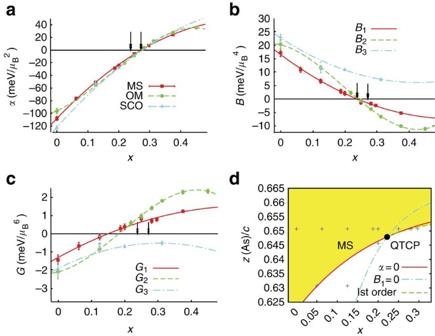Figure 3:Ab-initioLandau parameters. (a–c) Landau parameters for the three possible magnetic phases as function of the doping concentrationx. Dots are the numerical results whereas the lines are fits, as explained in the text. The left (right) arrow indicate the point whereB1=B2=0 (α=0). (d) LDA phase diagram for the MS in thez(As)-doping plane. The white region indicates the region of stability of the non-magnetic state. Crosses indicate the points where LDA constrained computations have been performed. Figure 3: Ab-initio Landau parameters. ( a – c ) Landau parameters for the three possible magnetic phases as function of the doping concentration x . Dots are the numerical results whereas the lines are fits, as explained in the text. The left (right) arrow indicate the point where B 1 = B 2 =0 ( α =0). ( d ) LDA phase diagram for the MS in the z (As)-doping plane. The white region indicates the region of stability of the non-magnetic state. Crosses indicate the points where LDA constrained computations have been performed. Full size image Figure 3b and c show the behaviour of the quartic and sixth-order Landau parameters as a function of the doping concentration x . The behaviour is rather smooth and can be simply captured assuming a quadratic polynomial expansion except for the OM where a cubic term becomes important far from the critical point. For the MS and the OM phases, we find that the quartic coefficient B of the Landau expansion becomes negative above x B =0.24< x α . Therefore, the transitions from the non-magnetic state to the MS and OM phase are of first order whereas for the SCO state, B 3 >0, and the transition is a conventional second-order one. One can judge the relevance of the QTCP in the thermal crossovers by computing the height of the energy barrier at the point in which the magnetic and non-magnetic solutions become degenerate. For the MS, the barrier from the fits is nominally ~2 K per Fe atom that is much below the limit of accuracy of the computation, thus for all practical propose, the MS-non-magnetic transition occurs at a QTCP in LDA. The low barrier reflects an almost vanishing metastability range around the transition and the physics will be dominated by QTCP behaviour. The OM state has a larger range of metastability (c.f. Fig. 4 ) but still with a negligible barrier at the transition point (~10 K). 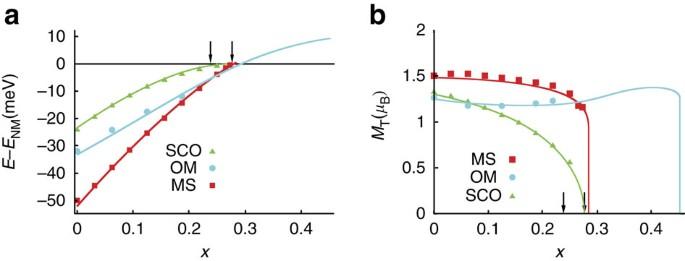Figure 4: Energy versus doping. (a) Energy per Fe and (b)MTin the unconstrained LDA (dots) and the Landau theory (lines). The left (right) arrow indicate the point whereB1=B2= 0 (α = 0). Figure 4: Energy versus doping. ( a ) Energy per Fe and ( b ) M T in the unconstrained LDA (dots) and the Landau theory (lines). The left (right) arrow indicate the point where B 1 = B 2 = 0 (α = 0). Full size image Figure 4a shows the energy of the different phases. The end of the line indicates the spinodal point, that is, the point at which the state disappears as a saddle-point solution of the Landau equations. The MS stripe is the most stable phase except close to the transition to the paramagnet where the OM phase becomes stable in a small doping interval. The OM preserves C 4 symmetry and has the same structure factor as an incoherent superposition of ( π , 0) and (0, π ) twins of the MS state, so it is difficult to distinguish with magnetic neutron scattering alone. It is interesting that for 122 compounds, a state with magnetic order but without detectable orthorhombicity has been reported [41] that can be taken as a signature of the OM state. Figure 4b shows M T versus doping. Despite the abrupt suppression of the order parameter from M T ~1 μ B to M T ≡0 for the MS, the transition is weakly first order. The OM magnetization shows a sharper first-order behaviour, although, as discussed above, the barrier is very small. The SCO behaves as a typical second-order transition. The behaviour of the order parameter of the MS is consistent with the sudden drop of the magnetization as a function of doping observed in this compound [35] . Such behaviour reinforces our conclusion that the system is close to a QTCP, although our critical doping is overestimated as discussed below. The fact that the OM state lies only less than 10 meV above the paramagnetic state for a large range of doping suggests that fluctuations to this state may be the most relevant ones in the superconducting region. Phase diagram The LDA critical doping ~0.26 is larger than the experimental one 0.05~0.06 in this compound. Because LDA neglects fluctuations, the derived Landau parameters should be considered as 'bare' parameters. One well-known effect of fluctuations is to reduce the stability of the ordered phases [42] , [43] shifting the critical doping in the correct direction. Also because of the small energies involved, the actual transition will be sensitive to details as the choice of the functional or changes due to the relaxation of the structure. In particular, it is known that the magnetism is very sensitive to z (As), the z coordinate of the As in the unit cell [37] , [38] , [44] , [45] . Relaxing z (As) results in a decrease of around 0.1 c ( c =0.87Å). We performed also computations with selected values of z (c.f. Fig. 2e ) and constructed the zero-temperature phase diagram shown in Figure 3d that shows the location of the QTCP in the z (As)-doping plane. We see that a decrease of z (As) indeed shifts the transition to the right range of doping moving from the weakly first-order region (right of the QTCP) to the second-order region. We also show the line B 1 =0. We see that, even if one takes a relaxed z and a smaller critical doping, still the transition is dominated by the proximity to this line. Indeed, we find that the B 1 coefficient depends weakly on z ( As ) c , so for doping x =0.05 and z/c =0.6307 we find B 1 ~10 meV/ μ B 4 . Taking a characteristic moment of M *~0.5 μ B this implies a negligible energy scale B 1 ( M *) 4 ~7 K that again points to anomalously soft magnetism due to proximity to the QTCP. A decrease in z ( As )/ c yields a substantial reduction of the total Fe magnetic moments towards the range observed in experiments [17] leading in the end to a consistent picture from the point of view of magnetization, critical doping and vicinity to the QTCP. The effects of fluctuations on a QTCP have been recently analysed in renormalization group studies [22] , [23] and within a phenomenological spin fluctuation theory [21] obtaining similar results. Applying the results of Misawa et al ., we obtain that the coefficient in the quartic term gets renormalized due to spin fluctuations as B 1 R = B 1 +15 KG 1 where K is the zero-temperature spin fluctuation term (corresponding to the average of the magnetic fluctuations near the ordering wavevector) and is expected to be of the order of a fraction of 1 μ B 2 . Because G 1 is generically small in the doping range of interest, this correction is expected to be not too large. In particular, near the critical doping x ~0.05 where G 1 <0, it decreases the magnitude of B 1, thereby driving the system even closer to the QTCP. It has been suggested [11] that the quantum phase transition in iron pnictides can be described by the effective long-wavelength field theory of a spin model with nearest- and next-nearest-neighbour antiferromagnetic couplings J 1 , J 2 . By introducing two Néel order parameters in different sublattices and , the second and fourth order terms of the effective Lagrangian can be recast as For α X <0, the field theory predicts an Ising order described in terms of an Hubbard-Stratonovich field linearly coupled to which is responsible for the lattice distortion experimentally observed in pnictides. We can determine whether the Ising symmetry is broken as the parameters of the field theory are related to our Landau coefficients by u = B 3 /2, γ 1 = B 2 – B 3 and α X = B 2 – B 1 . Increasing the doping, for the experimental atomic positions, α X changes from positive to negative at x B ( Fig. 3b ) immediately before the transition. Therefore, the Ising symmetry is restored before the magnetic order vanishes. This is consistent with the appearance of the OM state in a small doping interval as shown above. In addition, the smallness of α X implies a structural transition very close to the magnetic transition as a function of doping [11] which is consistent with the experimental phase diagram of doped LaOFeAs [35] . We have shown that magnetism in the iron-pnictide superconductor LaFeAsO 1− x F x is surprisingly close to a QTCP, and we have determined ab initio the coefficients of a Landau expansion around it. The energy landscape is anomalously flat close to the zero-temperature magnetic–non-magnetic transition giving rise to very soft behaviour of the order parameter in the sense that it can experience large changes as a result of weak perturbations. We believe frustration has an important role in this result as it tends to turn Stoner-like transitions into weakly first-order ones [30] . The degeneracy of the ground state close to a QCP is believed to boost superconductivity [3] , [16] . This effect should be enhanced close to a QTCP, where the degeneracy is even larger, and may have an important role in determining the high critical temperature of iron pnictides. It is interesting that Si and Abrahams have linked magnetic frustration and superconductivity [46] using a quite different point of view, namely a t-J-J′ model for iron-based superconductors. Similar to us, they argue that magnetic frustration accumulates entropy at low temperatures that is released by the superconducting order. Whereas we have focused on a 1111 compound, one expects similar behaviour to occur in 122 compounds. Experiments in undoped SrFe 2 As 2 and BaFe 2 As 2 have shown that externally applied pressure can quench magnetism leading to superconductivity with T c as high as 29 K [47] . Therefore, combination of pressure and doping or uniform magnetic fields would make experiments exactly at the QTCP possible, thereby elucidating the effect of this unusual critical behaviour on superconducting and normal state properties. In particular, the strong fluctuations of the order parameter close to the QTCP are expected to coexist with strong fluctuations of variables conjugate to the control field [21] , for example, strong fluctuations of the structure in a pressure-controlled experiment. Ab-initio computations LDA computations were performed using the Vienna ab-initio simulation package (VASP) [48] . The Kohn–Sham equations in the self-consistent calculations have been solved using the projector-augmented wave method [49] with the valence pseudo-wavefunctions expanded in a plane wave basis set with a cut-off energy of 500 eV. All the integrations in the Brillouin zone were performed initially with a Gaussian smearing method and then checked with a tetrahedron scheme [50] , using a sampling grid of 10×10×6 k-points. For iron pnictides, the method of choice is LDA because it provides magnetic properties closer to experiment than, for example, generalized gradient approximation [45] . We used experimental lattice and internal parameters fixed at zero doping [17] with symmetry group P4/nmm, constructing our unit cell with 4 Fe sites to be able to allocate the mentioned magnetic structures. The MS phase breaks C 4 symmetry, and thus a lattice distortion is expected, as observed experimentally. However, we were interested in the behaviour close to the QCP between the magnetic and non-magnetic state, where the orthorhombicity becomes negligible [51] . Therefore, this effect has been neglected for simplicity. We also performed calculations changing the z coordinate of the As as explained in the main text. Electron doping has been introduced in our computations by the virtual crystal approximation [52] . Constrained LDA We fixed both the modulus and direction of the magnetization to the patterns dictated by the Landau theory by performing constrained-LDA calculations [31] and computing the total energy as a function of M T . The local magnetic moments were found by integration of the magnetization density in atomic Wigner–Seitz spheres centred at the Fe sites. To implement the constraint we introduced a penalty energy quadratic in the difference between the LDA magnetization and the target magnetization with a large prefactor. Minimization of the new functional yields the LDA energy for the target magnetization with a negligible contribution of the penalty energy. The energyversus M T curves were fitted with expressions equation (1) to determine the Landau coefficients. The minimum of the Landau energy determines the equilibrium magnetization. How to cite this article: Giovannetti, G. Proximity of iron pnictide superconductors to a quantum tricritical point. Nat. Commun. 2:398 doi: 10.1038/ncomms1407 (2011).